Discovery of chlamydial peptidoglycan reveals bacteria with murein sacculi but without FtsZ Chlamydiae are important pathogens and symbionts with unique cell biological features. They lack the cell-division protein FtsZ, and the existence of peptidoglycan (PG) in their cell wall has been highly controversial. FtsZ and PG together function in orchestrating cell division and maintaining cell shape in almost all other bacteria. Using electron cryotomography, mass spectrometry and fluorescent labelling dyes, here we show that some environmental chlamydiae have cell wall sacculi consisting of a novel PG type. Treatment with fosfomycin (a PG synthesis inhibitor) leads to lower infection rates and aberrant cell shapes, suggesting that PG synthesis is crucial for the chlamydial life cycle. Our findings demonstrate for the first time the presence of PG in a member of the Chlamydiae . They also present a unique example of a bacterium with a PG sacculus but without FtsZ, challenging the current hypothesis that it is the absence of a cell wall that renders FtsZ non-essential. C hlamydiae are members of the Planctomycetes–Verrucomicrobia–Chlamydiae (PVC) bacterial superphylum [1] . Like most other bacteria, some PVC bacteria are already known to possess peptidoglycan (PG), that is, chains of alternating N-acetylglucosamine and N-acetylmuramic acid sugars crosslinked by short peptides. PVC bacteria also display striking eukaryote-like and archaea-like cell biological features, which have suggested intriguing hypotheses about their role in cellular evolution [2] , [3] . In Verrucomicrobia and almost all other bacteria, septal PG synthesis is orchestrated by the FtsZ cytoskeleton [4] , [5] . In contrast, Planctomycetes lack both PG and FtsZ [5] . This fits to the notion that PG-loss renders FtsZ dispensable, like in mycoplasmas [6] or L-form bacilli [7] . Although from genome sequences it is clear that chlamydiae do not possess FtsZ, the presence or absence of chlamydial PG has been highly controversial [8] , [9] , [10] , [11] , [12] , [13] , [14] , [15] , [16] . One early study reported the colorimetric detection of muramic acid in chlamydiae [14] , but more reliable chromatographic methods subsequently failed to confirm this result [11] , [15] . All attempts to purify chlamydial sacculi have failed [10] , [12] and no periplasmic density layers have been detected between the inner and outer membranes of chlamydiae by electron microscopy (EM) (including for instance [17] , [18] , [19] ). The apparent absence of PG in chlamydiae is surprising, however, as despite their highly reduced genomes, a nearly complete pathway for the synthesis of PG is present in the genomes of all chlamydiae [13] . In addition, several of the chlamydial PG biosynthetic enzymes have been characterized and shown to be functional in vitro and in complementation assays [20] , [21] , [22] , [23] , [24] , [25] . Here we look for the evidence of PG cell walls in two diverse and deeply rooting chlamydiae [26] , Protochlamydia amoebophila and Simkania negevensis . Through electron cryotomography (ECT), biochemical purification, enzymatic digestion, mass spectrometry (MS), fluorescence microscopy and antibiotic treatment, we show that P. amoebophila are indeed surrounded by sacculi containing a new type of PG. In contrast, no evidence of PG is found in S. negevensis . These results prove that some chlamydiae do in fact synthesize PG sacculi, explaining the presence of PG-synthetic genes, but raising new questions about the identity and purpose of the modifications and the mechanisms of cell division in the absence of FtsZ. ECT of the chlamydial cell envelope Two diverse and deeply rooting members of the chlamydial phylum, S. negevensis and P. amoebophila, were imaged by ECT in a near-native state. Bacteria were purified from amoeba cultures, plunge-frozen and 25 and 20 tomograms were collected of intact cells ( Fig. 1 ). Density profiles through the cell envelopes of the two species were quite different. Although four layers were resolved in Simkania envelopes ( Fig. 1b,c ), five layers were resolved in Protochlamydia ( Fig. 1e,f ). Because the individual leaflets of lipid bilayers can be resolved in some cryotomograms, especially when the images are taken close to focus, in the case of Simkania , it is unclear whether the four layers represent the two leaflets of the outer and inner membranes (‘O’ and ‘A’ being the two leaflets of the outer membrane, and layers ‘B’ and ‘I’ being the two leaflets of the inner membrane), or whether one or more of these layers are non-membranous. The facts that layers O and A have fairly similar contrast and are consistently spaced even through the undulations are consistent with them being two leaflets of a single (outer) bilayer membrane. Their separation (~5 nm), however, is much larger than typical phospholipid bilayer membranes, whose two density peaks (from the phospholipid head groups) are only 3.7–4 nm apart [27] . Similarly, Simkania layers B and I may be the two leaflets of a single (inner) membrane, as they have similar contrast and a consistent spacing, but again they appear too far apart. In contrast to the Simkania envelope, the profile of Protochlamydia surprisingly resembled those of other Gram-negative bacteria with two membranes and a PG cell wall [28] , [29] , [30] . Between the Protochlamydia outer and inner membranes (labelled ‘O’ and ‘I’, respectively) there appeared to be three additional layers (labelled ‘C’–‘E’). The similar-looking three layers in Treponema pallidum (from the outside in) were identified as proteinaceous (lipoproteins), PG and again proteinaceous [29] . By analogy this suggests that layer C is composed of lipoproteins (perhaps connecting the outer membrane to the cell wall) and other outer-membrane-associated proteins, layer D is a cell wall and layer E is composed of lipoproteins and inner-membrane-associated proteins (perhaps including the penicillin-binding proteins responsible for cell wall synthesis, the lipoprotein OmcA and the cysteine-rich protein OmcB). Although other interpretations remain possible (cysteine-rich disulphide-crosslinked envelope proteins have been suggested to be the functional equivalent of PG in chlamydiae [31] ), the most important and clear observation was that Protochlamydia exhibit a distinct periplasmic layer (D). 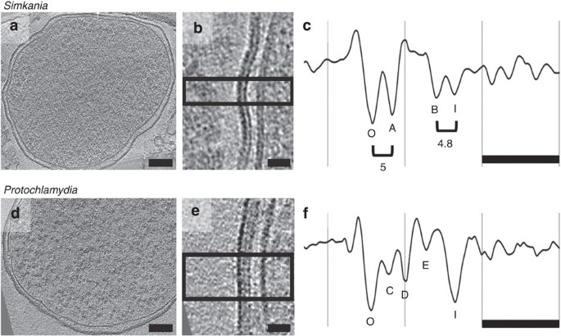Figure 1: Chlamydial cell envelopes are multi-layered. Simkania(a–c) andProtochlamydia(d–f) cells were purified from asynchronously infected amoeba cultures, plunge-frozen and imaged by ECT. Shown are tomographic slices through reticulate bodies (a,dandb,eenlarged) and corresponding density profiles (c,f) of the cell envelopes. Profiles are enlarged, aligned and cropped relative to the outer membrane. Distances between peaks (in nm) are indicated. In contrast to theSimkaniaprofile, theProtochlamydiaprofile resembles those of other bacteria with PG cell walls (see text for a full discussion of each profile and layer). Scale bar, 100 nm ina,dand 20 nm inb,c,e,f. Figure 1: Chlamydial cell envelopes are multi-layered. Simkania ( a – c ) and Protochlamydia ( d – f ) cells were purified from asynchronously infected amoeba cultures, plunge-frozen and imaged by ECT. Shown are tomographic slices through reticulate bodies ( a , d and b , e enlarged) and corresponding density profiles ( c , f ) of the cell envelopes. Profiles are enlarged, aligned and cropped relative to the outer membrane. Distances between peaks (in nm) are indicated. In contrast to the Simkania profile, the Protochlamydia profile resembles those of other bacteria with PG cell walls (see text for a full discussion of each profile and layer). Scale bar, 100 nm in a , d and 20 nm in b , c , e , f . Full size image Purification and imaging of sacculi In order to explore whether any of the observed periplasmic layers consisted of PG, we attempted to purify sacculi by boiling chlamydial cells (obtained from asynchronously infected amoeba cultures) in 4% sodium dodecyl sulphate. Strikingly, in three independent experiments, we observed sacculus-like structures in preparations from Protochlamydia ( Fig. 2a–d ), but not from Simkania (two experiments). Protochlamydia sacculi diameters (679 nm ±34 s.d. n =10) and morphologies matched the size and shape of intact cells. Protochlamydia sacculi had one or two 5–7 nm thick layers (arrowheads in Fig. 2e ), plus mesh-like (up to 30 nm long) high-density aggregates attached to the outside (arrows in Fig. 2d ). 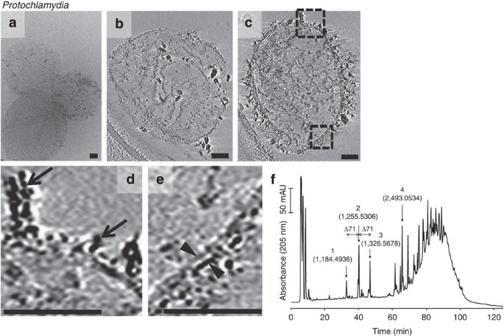Figure 2:Protochlamydiasynthesize purifiable sacculi that contain PG. Cryoprojections (a) and tomographic slices (b–e) through sacculi-like structures purified fromProtochlamydiacells. We were unable to obtain similar structures fromSimkania. Sacculi had one or two layers (arrowheads) plus short high-density filaments (arrows) on the outside (cenlarged ind,e). Sacculi were digested, reduced and separated by HPLC (f). MS analysis of peaks 1–3 (neutral masses indicated in Da) indicated the presence of modified PG (see alsoTable 1andSupplementary Fig. S1). Scale bars, 100 nm. Figure 2: Protochlamydia synthesize purifiable sacculi that contain PG. Cryoprojections ( a ) and tomographic slices ( b – e ) through sacculi-like structures purified from Protochlamydia cells. We were unable to obtain similar structures from Simkania . Sacculi had one or two layers (arrowheads) plus short high-density filaments (arrows) on the outside ( c enlarged in d , e ). Sacculi were digested, reduced and separated by HPLC ( f ). MS analysis of peaks 1–3 (neutral masses indicated in Da) indicated the presence of modified PG (see also Table 1 and Supplementary Fig. S1 ). Scale bars, 100 nm. Full size image Digestion and biochemical analyses of sacculi To check for the presence of PG in the purified sacculi, we digested the samples with cellosyl, a glycan strand-cleaving PG muramidase. Cellosyl released soluble material from insoluble sacculi, which was reduced with sodium borohydride and analysed by high-pressure liquid chromatography (HPLC) using conditions for separating muropeptides [32] . The chromatogram ( Fig. 2f ) showed three main peaks in the monomeric region (20–50 min) and many peaks after 60 min that are poorly separated at higher retention time (>75 min) forming a ‘hump’, which is typical for highly crosslinked and/or incompletely digested PG material [33] . The retention times and overall pattern of cellosyl digestion products were different, however, from those of muropeptide mixtures obtained from other Gram-positive and Gram-negative bacteria. To characterize this material, the three main cellosyl products in the monomeric region and one well-separated main product at the beginning of the ‘hump’ region were analysed by MS. The determined neutral masses of the earlier three products were higher than what would be expected for monomeric muropeptides, but the masses of products 1 and 2 and of products 2 and 3 both differed by 71 Da, a typical feature of monomeric muropeptides with a tri-, tetra- and pentapeptide, respectively, due to the presence of none, one or two D -alanine residues ( Fig. 2f ). In MS/MS analysis, the three products were fragmented in a similar way, showing that they are related ( Supplementary Fig. S1 , Table 1 ). For all three peaks, we observed mass differences to the parent ion corresponding to the loss of Glc N Ac, Glc N AcMur N Ac(r) (r, indicates reduction to N -acetylmuramitol), Glc N AcMur N Ac(r)- L -alanine and Glc N AcMur N Ac(r)- L -alanine- D -glutamate, confirming that products 1–3 are all muropeptides. The neutral masses of the Protochlamydia products 1, 2 and 3 were all 314.12 Da larger than the masses of the reduced monomeric muropeptides (with tri-, tetra- or pentapeptide) from Gram-negative bacteria [34] , however, suggesting the presence of a common modification in the Protochlamydia muropeptides. The neutral mass of product 4 was consistent with a peptide crosslinked dimer of product 2. Additional mass differences that occurred in all fragmentation spectra indicated the presence of the same and as yet unknown modifications with 129 and 203 Da, respectively, explaining the higher mass of Protochlamydia muropeptides 1–3 compared to the monomeric muropeptides of Escherichia coli . Table 1 Fragmentation masses from fractions of reduced P. amoebophila muropeptides. Full size table To confirm that PG was a major component of Protochlamydia sacculi and check for the presence of disulphide-crosslinked protein components, purified sacculi were subjected to lysozyme and dithiothreitol treatment, respectively, and imaged with negative stain EM. Only the incubation with lysozyme degraded the sacculi ( Supplementary Fig. S2 ). Fluorescence imaging of D -alanine incorporation in vivo To further confirm the presence of PG in Protochlamydia sacculi, we tested whether fluorescently labelled amino acids (fluorescent D -amino acids (FDAA); labelled D -alanine in our experiments) [35] would be incorporated into chlamydial cells in vivo . Incubation of amoeba cultures continuously infected with Protochlamydia (including reticulate bodies, elementary bodies and transitional stages) with FDAA (HADA (hydroxy coumarin-carbonyl-amino- D -alanine) and BADA (4,4-difluoro-5,7-dimethyl-4-bora-3a,4a-diaza-s-indacene-3-propionic acid-3-amino- D -alanine)) resulted in multiple strong and chlamydial cell-sized signals inside amoeba cells ( Fig. 3a–d , Supplementary Fig. S3 ). In many cases, the FDAA labelling in infected amoebae overlapped with staining of the chlamydial cells by 4′,6-diamidino-2-phenylindole (DAPI) or chlamydiae-specific fluorescence in situ hybridization (FISH). Not all cells stained by FISH/DAPI showed a corresponding FDAA signal, at least in part because chlamydial cells were in different developmental stages, including non-replicating elementary bodies. No signals were detected when uninfected amoebae were incubated with FDAA ( Supplementary Fig. S3D, E ), or when infected amoebae were incubated with dimethylsulphoxide only. Interestingly, purified Protochlamydia elementary bodies (which cannot undergo cell division and are therefore probably not actively synthesizing new PG) also did not show labelling upon incubation with FDAA ( Supplementary Fig. S3B,C ), indicating that PG synthesis takes place during Protochlamydia replication inside the host. Amoeba cultures infected with Simkania , on the other hand, showed either no signals (using BADA) or signals similar to the background level (using HADA) upon labelling with FDAA ( Supplementary Fig. S4A,B ), consistent with the absence of purifiable sacculi. Purified Simkania cells were not labelled by either dye ( Supplementary Fig. S4C,D ). 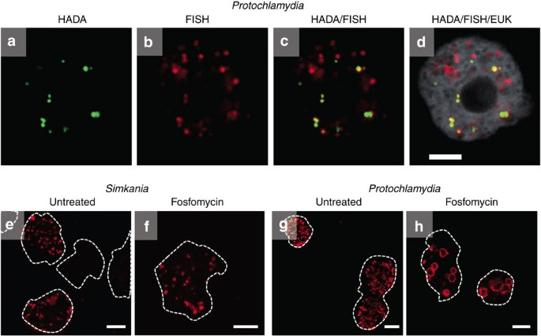Figure 3:ProtochlamydiaincorporateD-alaninein vivoand are sensitive to fosfomycin. Protochlamydia-infected amoebae (a–d), but not purifiedProtochlamydiacells (Supplementary Fig. S2) or uninfected amoeba cells (Supplementary Fig. S2), stained positively for new PG synthesis with fluorescently labelledD-alanine dyes HADA (a) and BADA (Supplementary Fig. S2), confirming the synthesis of PG in actively growingProtochlamydia. Specific FISH staining of chlamydial cells (b, overlay withashown inc) and the eukaryotic host (d, shows overlay withc) are shown. The treatment ofProtochlamydia-infected amoeba cultures (amoeba cell outlines in white) with cell-wall-synthesis-targeting fosfomycin (h, control shown ing) resulted in a dramatic decrease in infection rate and aberrant or larger chlamydial cell shapes (shown are immunofluorescent stainings of chlamydial outer membrane proteins), suggesting a crucial role of PG in theProtochlamydialife cycle. Fosfomycin did not affectSimkania(f, control shown ine). Scale bars, 5 μm ind, 10 μm ine–h. Figure 3: Protochlamydia incorporate D -alanine in vivo and are sensitive to fosfomycin. Protochlamydia -infected amoebae ( a – d ), but not purified Protochlamydia cells ( Supplementary Fig. S2 ) or uninfected amoeba cells ( Supplementary Fig. S2 ), stained positively for new PG synthesis with fluorescently labelled D -alanine dyes HADA ( a ) and BADA ( Supplementary Fig. S2 ), confirming the synthesis of PG in actively growing Protochlamydia . Specific FISH staining of chlamydial cells ( b , overlay with a shown in c ) and the eukaryotic host ( d , shows overlay with c ) are shown. The treatment of Protochlamydia -infected amoeba cultures (amoeba cell outlines in white) with cell-wall-synthesis-targeting fosfomycin ( h , control shown in g ) resulted in a dramatic decrease in infection rate and aberrant or larger chlamydial cell shapes (shown are immunofluorescent stainings of chlamydial outer membrane proteins), suggesting a crucial role of PG in the Protochlamydia life cycle. Fosfomycin did not affect Simkania ( f , control shown in e ). Scale bars, 5 μm in d , 10 μm in e – h . Full size image Protochlamydia sensitivity to cell-wall-targeting antibiotics Owing to the high conservation of PG throughout the bacterial domain of life, many antibacterial drugs target PG synthesis. The so-called chlamydial anomaly [16] is that despite the fact that PG has not been detected in pathogenic chlamydiae, these organisms are sensitive to cell-wall-targeting β-lactam antibiotics. Penicillin, for instance, leads to the formation of enlarged aberrant cells [36] , [37] and blocks the conversion between developmental stages [38] . Environmental chlamydiae, in contrast, are resistant to β-lactams [39] , [40] –possibly due to putative β-lactamases encoded in their genomes. To explore the role of the PG sacculus in the Protochlamydia life cycle, we used an alternative PG synthesis-targeting antibiotic (fosfomycin) to treat infected amoeba cells. The addition of 500 μg ml −1 fosfomycin to Protochlamydia -infected amoeba cultures led to a significant decrease in infection rate (20.2%±8 infected amoebae for fosfomycin-treated cultures versus 95.8%±2.2 infected amoebae for untreated cultures; P <0.0001, unpaired t -test). Protochlamydia cells within treated cultures were also up to eight-times larger than normal (diameters of up to 6 μm) ( Fig. 3g,h ). Lower fosfomycin concentrations (25 μg ml −1 and 100 μg ml −1 ) induced the formation of fewer aberrant forms and did not affect the infection rate (not shown). Fosfomycin treatment of Simkania -infected amoeba cultures led to only a slight decrease in infection rate (59.9%±5.6 infected amoebae for fosfomycin-treated cultures versus 67%±1.7 infected amoebae for untreated cultures) and no differences in cell size were detected ( Fig. 3e,f ). We conclude that Protochlamydia synthesize sacculi containing PG that can be hydrolysed by cellosyl, contains monomeric and crosslinked muropeptides, and carries yet unknown modifications at virtually every subunit. No evidence of PG in Simkania was found. Fluorescence imaging of D -Ala incorporation in vivo and monitoring of cell wall antibiotic sensitivity further suggested that the Protochlamydia PG sacculus has an important role in cell cycle and shape. This challenges previous speculations that chlamydiae synthesize a small ring of PG only during cell division [41] . Because this might still be true for Simkania and pathogenic chlamydiae, however, our data prompts a reconsideration of whether these organisms lack PG entirely (and the effects of β-lactams are pleiotropic) or if they synthesize novel PG structures that are not purified by standard sacculus preparation protocols. The presence of sacculi in Protochlamydia but not in Simkania matches the less complete set of synthetic genes in the latter: Simkania , as well as pathogenic chlamydiae, lack an undecaprenyl-diphosphate phosphatase (UppP) and alanine/glutamine racemases (Alr, MurI) ( Supplementary Table S1 ) [13] , [42] , [43] . Interestingly, transglycosylases have not been found in any chlamydial genomes ( Supplementary Table S1 ) [13] or in the genomes of a few other PG-possessing bacteria [44] , [45] , so some other enzyme(s) must be capable of synthesizing glycan strands. The presence of PG sacculi in Protochlamydia and in the Chlamydiae ’s sister phylum Verrucomicrobia [46] , together with the fact that the more basal chlamydial lineages have more complete PG synthesis pathways make it likely that the last common chlamydial ancestor synthesized a PG sacculus. The detection of a PG-containing sacculus in Protochlamydia challenges the view that FtsZ is essential in PG-possessing bacteria [4] , [6] , [7] , however, because to our knowledge, Protochlamydia is the first example of a bacterium with a PG cell wall, but without FtsZ. Studying cell division and septal development in this organism could help clarify the role of FtsZ and the evolutionary transition to PG- and FtsZ-independency. Cultivation of organisms Acanthamoeba castellanii Neff infected with P. amoebophila UWE25, or A. castellanii UWC1 infected with S. negevensis , were cultivated in TSY medium (30 g l −1 trypticase soy broth, 10 g l −1 yeast extract, pH 7.3) at 20 °C. Amoebal growth was monitored by light microscopy and medium was exchanged every 3–6 days. The presence and identity of the chlamydial symbionts was verified by isolation of DNA from cultures followed by amplification and sequencing of the 16S rRNA genes. In addition, FISH using specific probes combined with DAPI staining of infected cultures was performed using specific probes for the respective symbiont [47] . Amoebae infected with chlamydiae were allowed to attach on slides and were fixed with 4% formaldehyde at 20 °C. Cells were hybridized for 1.5 h at 46 °C at a formamide concentration of 25% with the Protochlamydia -specific probe E25-454 (5′-GGA TGT TAG CCA GCT CAT-3′) or the Simkania -specific probe Simneg-183 (5′-CAG GCT ACC CCA GCT CTC-3′) and the probe EUB338 (ref. 48 ). Subsequently, cells were stained with DAPI (0.5 μg ml −1 in PBS) for 5 min, and slides were analysed using an epifluorescence microscope. Purification of chlamydiae Infected A. castellanii cultures were harvested by centrifugation (7,197 × g , 10 min), washed in Page’s Amoebic Saline (PAS) [49] , centrifuged and resuspended in PAS. Amoeba cells were disrupted by vortexing with an equal volume of glass beads for 3 min. Glass beads and cell debris were removed by centrifugation (5 min, 300 × g ). The supernatant was filtered through a 1.2 μm filter and centrifuged at maximum speed for 10 min, 18,000 × g. The obtained pellet was resuspended in PAS. Plunge-freezing For plunge-freezing, copper/rhodium EM grids (R2/2 or R2/1, Quantifoil) were glow-discharged for 1 min. A 20 × -concentrated bovine serum albumin-treated solution of 10 nm colloidal gold (Sigma) was added to purified chlamydiae or sacculi (1:4 v/v) immediately before plunge freezing. A 4-μl droplet of the mixture was applied to the EM grid, then automatically blotted and plunge-frozen into a liquid ethane–propane mixture [50] using a Vitrobot (FEI Company) [51] . Electron cryotomography Images were collected using a Polara 300 kV FEG transmission electron microscope (FEI Company) equipped with an energy filter (slit width 20 eV; Gatan) on a lens-coupled 4 k × 4 k UltraCam CCD (Gatan). Pixels on the CCD represented 0.95 nm (22,500 × ) or 0.63 nm (34,000 × ) at the specimen level. Typically, tilt series were recorded from −60° to +60° with an increment of 1° at 10 μm under-focus. The cumulative dose of a tilt-series was 180–220 e − /Å 2 . UCSF Tomo [52] was used for automatic acquisition of tilt-series and 2D projection images. Three-dimensional reconstructions were calculated using the IMOD software package [53] or Raptor [54] . Tomograms were visualized using 3dMOD [53] . Density profiles were generated using ImageJ. Fluorescent labelling of PG Newly synthesized PG was labelled using FDAA [35] . A. castellanii cells continuously infected with Protochlamydia or Simkania were harvested and resuspended in a mixture of TSY and PAS (1:1). Cells were incubated with 1.5 mM HADA [35] or BADA for 6 h with gentle shaking. Cells were pelleted, washed three times and fixed with 4% formaldehyde followed by FISH using the chlamydia-specific probe Chls-0523 or DAPI-staining. As a control, uninfected amoebae and purified chlamydiae were treated in the same way. Antibiotic treatment of infected amoeba cultures A. castellanii were seeded into the wells of a multi-well dish and infected with purified Simkania and Protochlamydia elementary bodies [55] . After centrifugation at 600 × g for 10 min, the medium was exchanged for TSY supplemented with fosfomycin (0, 25, 100 or 500 μg ml −1 , respectively). Medium was exchanged once at 48 h post infection. Cells were fixed with methanol at 96 h post infection followed by immunofluorescence analysis using either anti-PomS antibodies [55] or anti- Simkania antibodies raised against purified chlamydiae. The number of infected amoebae was counted for each treatment. Preparation and composition analysis of sacculi Chlamydial cells were purified from 1.8 l ( Protochlamydia ) and 3 l ( Simkania ) of infected amoeba culture and, depending on the amount of harvested cells, resuspended in 2.6–5.2 ml 4% SDS (w/v). After shipping (overnight, room temperature), the suspensions were dripped into 4% SDS (preheated to 90 °C, 6 ml final volume) and stirred for 2.5 h at 90 °C. Sacculi were pelleted (30 min, 135,000 × g) in a TLA-100.3 rotor (Beckman Coulter), washed 4 × in 3 ml water, resuspended in 150 μl water and supplemented with 0.02% (w/v) sodium azide. Muropeptides were released from the PG by an overnight incubation with the muramidase Cellosyl (Hoechst, Frankfurt am Main, Germany) on a thermal shaker at 37 °C and 800 rpm. The sample was boiled for 10 min and centrifuged for 10 min at 13,500 × g . The muropeptides present in the supernatant were reduced with sodium borohydride and separated on a 250 × 4.6 mm 3-μm Prontosil 120-3-C18 AQ reversed phase column (Bischoff, Germany) at 55 °C using a 135 min gradient from 50 mM sodium phosphate pH 4.31 to 75 mM sodium phosphate pH 4.95, 15% methanol and a flow rate of 0.5 ml min −1 (ref. 32 ). Muropeptides were detected at 205 nm. Fractions were collected, concentrated in a SpeedVac, acidified by 1% trifluoroacetic acid and analysed by offline electrospray MS on a Finnigan LTQ-FT mass spectrometer (ThermoElectron, Bremen, Germany) in positive ion mode using mass scans over the mass range from m / z =300 to m / z =1,900 at a typical spray voltage of 1.1–1.5 kV [34] . Parent ion scans were acquired with an FT MS resolution setting of 100,000 (at m / z =400) with a typical mass accuracy of 3 ppm. MS/MS scans were performed in the ion trap, which has a typical mass accuracy for the fragment ion of±0.3 Da. MS spectra were deconvoluted to generate uncharged masses using the QualBrowser program (ThermoElectron, Bremen, Germany) [34] . Negative-stain EM of treated sacculi preparations Purified sacculi were incubated at 37 °C for 12 h in 20 μl total volume with either lysozyme (10 mg ml −1 ), dithiothreitol (5 mM) or phosphate buffered saline. Samples were applied to a Formvar-coated, carbon-coated, glow-discharged copper EM grid (Electron Microscopy Sciences). Samples were aspirated, stained with 1.5% uranylacetate and imaged on an FEI Tecnai T12 electron microscope. How to cite this article: Pilhofer, M. et al. Discovery of chlamydial peptidoglycan reveals bacteria with murein sacculi but without FtsZ. Nat. Commun. 4:2856 doi: 10.1038/ncomms3856 (2013).